Photo-switchable molecular monolayer anchored between highly transparent and flexible graphene electrodes A molecular ultra-thin film (for example, a molecular monolayer) with graphene electrodes would allow for the realization of superior stable, transparent and flexible electronics. A realistic prospect regarding the use of graphene in two-terminal molecular electronic devices is to fabricate a chemically stable, optically transparent, mechanically flexible and molecularly compatible junction. Here we report on a novel photo-switchable molecular monolayer, one side chemically and the other side physically anchored between the two graphene electrodes. The photo-switchable organic molecules specified with an electrophilic group are chemically self-assembled into a monolayer on the graphene bottom electrode, while the other end is physically contacted to the graphene top electrode; this arrangement provides excellent stability for a highly transparent and flexible molecular monolayer device with a high device yield due to soft contacts at the top electrode interface. Thus, the transparent graphene electrodes allow stable molecular photo-switching due to photo-induced changes in the molecular conformational length. One of the goals of molecule-based organic electronics is the realization of molecular functionalities in miniaturized and flexible electronic devices. Over the last few decades, numerous molecules have been suggested as viable candidates for such applications because of their electronically active or passive properties at the nanometre scale [1] , [2] , [3] , [4] . Fabrication processes for soft and stable contact to single molecules or molecular monolayers, and reliable measurements of the electronic properties of molecules, have been investigated. Recently, stabilised fabrication methods using soft conducting layers [5] , [6] , [7] were developed for device miniaturization using molecules. Miniaturization using molecules has also been explored via microscopic and spectroscopic studies of single molecules and molecular monolayers [8] , [9] , [10] , [11] . Realistic organic electrodes that are conductive, flexible and even transparent should form ideal contacts to a molecular monolayer of organic molecules in two-terminal crossbar devices and should ultimately be compatible with current standard electronic circuitry. To date, however, such characteristics have not been reported for molecular monolayer-integrated transparent and flexible electronics. As an intrinsically transparent, conductive and flexible electrode that allows for a photo-switchable molecular device, two-dimensional graphene is much more compatible with complementary metal-oxide semiconductor technology compared with other conductive carbon materials (for example, one-dimensional carbon nanotubes or zero-dimensional fullerenes). Graphene [12] , [13] , as a building block on a surface, allows for the one-sided grafting of aryl diazonium molecules via a well-known dediazoniation process [14] for sp 2 carbon network materials; this process is one of a few chemical reactions used to functionalise the graphene basal plane [15] . Aryl diazonium molecules spontaneously and thermally generate active aromatic radicals that create a carbon-carbon bond on the graphene surface. A large-area uniform molecular monolayer is subsequently formed. For two-terminal crossbar molecular devices, chemically grafting molecules (or assembly) on graphene electrode surfaces can produce a large contact area in the form of a molecular monolayer and amplify the signal of specific activities on the molecular scale. At the same time, the other side of the molecular monolayer is physically contacted to the graphene top electrode. Therefore, it is expected that the chemical attachment of single molecules to the graphene bottom electrode will completely prevent the local movement of molecules. In addition, the physical contact between the molecular monolayer and the graphene top electrode allows for a high bending angle with high bending cycles, and aids in preventing an electrical short, leading to transparent and highly flexible two-terminal crossbar molecular monolayer junctions with a high device yield. Herein, we report on a photo-switchable molecular monolayer between highly flexible and transparent graphene electrodes. The photo-switchable organic molecules are chemically self-assembled into a monolayer on the graphene bottom electrode, while the other end is physically contacted to the graphene top electrode. The arrangement of the graphene top electrode/physical contact/molecular monolayer/chemical contact/the graphene bottom electrode provides excellent stability for a transparent and flexible molecular monolayer device. Operation performances of graphene/photo-switching molecular monolayer/graphene devices are stable under severe mechanical stress conditions (for example, bending and twisting) and a large number of photo-switching cycles. Molecular monolayer with two-terminal graphene electrodes In this study, for two-terminal transparent and flexible graphene-based vertical molecular devices, novel aryl molecular monolayer tunnelling junctions between the two graphene electrodes were constructed ( Fig. 1a ). For transparent and flexible graphene-molecular monolayer–graphene junctions, aryl alkanes, as a passive molecular resistor, and aryl azobenzene, as a photo- and electro-active molecular switch, were carefully designed, and plastic substrates (for example, polydimethylsiloxane (PDMS) and polyethyleneterephthalate (PET)) were applied. For device preparation, large-area single-layer graphene grown on Cu foils through a chemical vapour deposition (CVD) process was carefully transferred onto the plastic substrates using the poly (methyl methacrylate) (PMMA)-mediated transfer method [16] . PDMS spin-coated on the PET substrate was introduced to reduce the surface roughness, which is an important step in increasing the device yield (over 80%). The aryl diazonium compounds (Methods and Supplementary Figs S1–S2 ) were self-assembled onto the graphene bottom electrode/substrate. The graphene top electrode was then transferred onto the aryl molecular monolayer/graphene/substrate in the same manner as the graphene bottom electrode ( Fig. 1a , Supplementary Note 1 , and Supplementary Figs S3–S6 ). Through electrophilic diazonium reactions, the band structures of the graphene electrodes are modulated such that covalent C-C sp [3] bonds form between the aryl radicals and C=C sp 2 carbon atoms. Electronic coupling between the graphene and molecules through covalent bonding may reduce the contact resistance [17] , thereby facilitating true molecular effects in monolayer-based devices. The energy positions of molecular tunnelling barriers between graphene electrodes with no applied bias are depicted ( Fig. 1b ), based on band diagrams of the two graphene sheets parallel located using a well-known band structure of graphene that has no band gap [18] . The formation of covalent C-C sp 3 bonds may induce the bandgap opening of the graphene electrode and reduce molecular tunnelling barriers ( Fig. 1c ). Molecular photo-switching induces a decrease (or increase) in the barrier height ( Fig. 1d ). In addition, the molecular tunnelling barriers are modified with the voltage applied to the two-terminal electronic devices ( Fig. 1e ), which characterizes molecular functionalities. 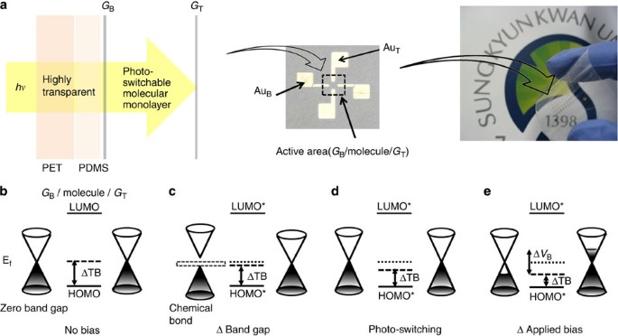Figure 1: Molecular monolayer devices with graphene-molecule-graphene structure. (a) Schematic of the structure of a vertical junction, an optical image of one device and an array of 100 devices on plastic. (b−d) Tunnelling barrier (ΔTB) corresponding to (b) a molecular barrier at zero bias, (c) a change in the graphene work function with diazonium reactions, (d) a change in a molecular barrier with photo-switching and (e) an applied bias (ΔVB/GB−GT). Molecular orbitals are denoted with HOMO (highest occupied molecular orbital) and LUMO (lowest unoccupied molecular orbital) at no bias and HOMO* and LUMO* after changing in a molecular barrier. Figure 1: Molecular monolayer devices with graphene-molecule-graphene structure. ( a ) Schematic of the structure of a vertical junction, an optical image of one device and an array of 100 devices on plastic. ( b − d ) Tunnelling barrier (ΔTB) corresponding to ( b ) a molecular barrier at zero bias, ( c ) a change in the graphene work function with diazonium reactions, ( d ) a change in a molecular barrier with photo-switching and ( e ) an applied bias (Δ V B / G B − G T ). Molecular orbitals are denoted with HOMO (highest occupied molecular orbital) and LUMO (lowest unoccupied molecular orbital) at no bias and HOMO* and LUMO* after changing in a molecular barrier. Full size image A certain amount of self-assembled aryl diazonium compounds on the graphene electrode (specifically 1-phenyloctane (N 2 + -PhC8), 1-phenyldecane (N 2 + -PhC10), 1-phenyldodecane (N 2 + -PhC12) and aryl azobenzene (N 2 + -PhC10AB) diazonium salts, which resulted in monolayers of PhC8, PhC10, PhC12 and PhC10AB, respectively) was quantitatively measured by a nanogravimetry technique using a graphene-covered quartz crystal resonator. The graphene-covered electrode ( Fig. 2a ) was pretested by atomic force microscopy (AFM) and cyclic voltammetry. The cyclic voltammograms ( Fig. 2b ) revealed that graphene perfectly blocked the adsorption/desorption of sulphate ions on gold and the oxidation/reduction of gold, which can limit the adsorption of aryl diazonium molecules on the backbone framework of graphene. 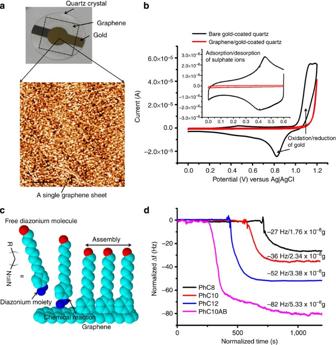Figure 2: Characterization of the grafting of aryl diazonium salts on graphene. (a) Photographic and AFM images (scale bar, 700 nm) of graphene completely covering the quartz crystal resonator (graphene/gold/quartz crystal). (b) Schematic of the process of molecular monolayer formation on graphene. (c) Cyclic voltammograms of bare gold-coated quartz (black line) and graphene/gold-coated quartz (red line) in 0.05 M H2SO4at a scan rate of 50 mV s−1. (d)In-situfrequency changes due to the self-assembly of aryl diazonium molecules. Figure 2c depicts the self-assembly process of aryl diazonium molecules on the graphene electrode. In-situ frequency changes show a dependency on the molecular mass ( Fig. 2d ). An average of 6.8±1.4 × 10 13 grafted molecules (on the surface area of 0.28 cm 2 ) was obtained, indicating that one in nine carbon atoms in the C=C sp 2 framework was occupied by an aryl molecule ( Supplementary Note 2 ). The characteristics of the aryl alkane monolayer on graphene were clearly identified ( Supplementary Figs S7–S9 ): (1) AFM topographical images and line profiles confirmed the molecular length of the aryl monolayer on the graphene ( Supplementary Fig. S7 ). (2) A transmission electron microscopy image revealed an expanded lattice constant due to the formation of sp 3 C-C bonds ( Supplementary Fig. S8 ). (3) The fourier transform infrared absorption peak of the sp 3 C–H stretching of the alkyl chain was identified and a Raman shift in the structural defects band appeared because of the generation of sp 3 carbon bonds ( Supplementary Fig. S9 ). Figure 2: Characterization of the grafting of aryl diazonium salts on graphene. ( a ) Photographic and AFM images (scale bar, 700 nm) of graphene completely covering the quartz crystal resonator (graphene/gold/quartz crystal). ( b ) Schematic of the process of molecular monolayer formation on graphene. ( c ) Cyclic voltammograms of bare gold-coated quartz (black line) and graphene/gold-coated quartz (red line) in 0.05 M H 2 SO 4 at a scan rate of 50 mV s −1 . ( d ) In-situ frequency changes due to the self-assembly of aryl diazonium molecules. 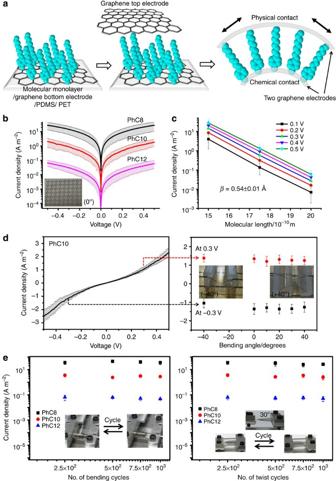Figure 3: Device characteristics of graphene-aryl alkane monolayer–graphene. (a) Schematic of a transparent and flexible molecular monolayer junction between the two graphene electrodes. (b) Current density-voltage plots on a log scale for each aryl alkane monolayer, inset: optical image of devices in an array; current density plots were generated from average values obtained from over 50 devices (the error bars denote the s.d. values). (c) Plots of the current density on a log scale at different voltages versus the molecular length in the aryl alkane monolayers. (d) Plots of the current density for a PhC10 monolayer as a function of bending angle upon bending the substrate to −40° and setting the current density at −0.3 V and 0.3 V; (inset) optical images of the substrates bent at −40° and 40°. (e) Preservation of the current density at −0.3 V against bending and twist cycling; current density plots were generated from average values obtained from over 15 devices (the error bars denote the s.d. values); (inset) optical images of substrate bending (Supplementary Movie 1) and twisting (Supplementary Movie 2) in a cycle. Full size image Electronic characteristics of molecular monolayers Figure 3a depicts the fabrication process and the stable performances of the graphene-aryl alkane-graphene vertical junctions to mechanical stresses. Plots of the electronic characteristics of the devices show that each molecular current density is inversely dependent on the molecular length ( Fig. 3b ). As expected, the grafted aryl alkanes (for example, PhC8, PhC10 and PhC12), a passive component in the circuit, behaved as molecular resistors. Our devices have the symmetric work function of the top and bottom electrodes with the asymmetric contacts that have one side chemically bound and the other side physically bound. The chemical contacts should have a higher junction conductance than the physical contacts [17] , [19] . However, differences in electrode work function and applied bias more effectively influenced changes in tunnelling barrier in molecular junctions, relative to the asymmetric effect of one- or two-sided chemically bound contacts [17] , [19] . Therefore, as shown in Fig. 3b , molecular junctions of both one- or two-sided chemically bound contacts with the same electrode material exhibit nearly symmetric current-voltage characteristics. The shortest aryl alkane (PhC8) provided the highest current density ( Fig. 3b ) among the three aryl alkanes, effectively lowering the current density of the graphene–graphene device without a molecular layer ( Supplementary Fig. S10 ). The current density exponentially decreased as the molecular length of the aryl alkanes increased, thus revealing the tunnelling mechanism [9] , [20] . Current density ( J ) plots obtained at several biases as a function of the molecular length ( d ) are described by the expression J exp(− βd ), where β is the tunnelling decay coefficient. The average β -value obtained was 0.54±0.01 Å −1 ( Fig. 3c ), which is lower than that for tunnelling transport through the aliphatic alkyl chains in n -alkanethiol/Au junctions [6] , [17] , [21] . This result confirms that the new junction system of graphene-molecule-graphene works reliably to obtain molecular tunnelling transport properties through molecular monolayers. Through bending tests, plots of the average current density at low voltages for graphene-PhC10-graphene devices as a function of the strain induced at the external bending angles (−40°~+40°) were obtained at −0.3 and 0.3 V ( Fig. 3d ). The graphene-PhC10-graphene devices featuring PhC8 and PhC12 did not exhibit a significant change even at different angles. Furthermore, for over 1,000 bending and twisting cycles, almost no change in the current density plots was observed at −0.3 V ( Fig. 3e ), which implies excellent device stability to the mechanical stresses. Figure 3: Device characteristics of graphene-aryl alkane monolayer–graphene. ( a ) Schematic of a transparent and flexible molecular monolayer junction between the two graphene electrodes. ( b ) Current density-voltage plots on a log scale for each aryl alkane monolayer, inset: optical image of devices in an array; current density plots were generated from average values obtained from over 50 devices (the error bars denote the s.d. values). ( c ) Plots of the current density on a log scale at different voltages versus the molecular length in the aryl alkane monolayers. ( d ) Plots of the current density for a PhC10 monolayer as a function of bending angle upon bending the substrate to −40° and setting the current density at −0.3 V and 0.3 V; (inset) optical images of the substrates bent at −40° and 40°. ( e ) Preservation of the current density at −0.3 V against bending and twist cycling; current density plots were generated from average values obtained from over 15 devices (the error bars denote the s.d. values); (inset) optical images of substrate bending ( Supplementary Movie 1 ) and twisting ( Supplementary Movie 2 ) in a cycle. Full size image Photo-switching operation of aryl azobenzene monolayers Molecular photo-switching in a graphene-aryl azobenzene monolayer–graphene junction was characterized by conformational structure-dependent molecular tunnelling behaviours ( Fig. 4 ). Photo-switching between the cis and trans isomers of aryl azobenzene molecules was pretested by ultraviolet-Vis spectroscopy ( Fig. 4a ). The junction was expected to behave as a molecular switch with light irradiation ( Fig. 4b–d ). Through the transparent graphene top window ( Supplementary Fig. S11 , as well as through the graphene bottom window), the light-driven structural transformation of azobenzene molecular monolayers was reversibly induced [22] . We found that the photo-switching operation of aryl azobenzene monolayers between the two graphene electrodes required longer irradiation time (for example, 45 min) than that of aryl azobenzene molecules in solution (for example, 30 min), presumably due to steric hindrance induced by the graphene top electrode even though the physical top contact should effectively allow for switching between trans and cis configurations. Current density plots of the aryl azobenzene monolayers (for example, PhC10AB) in the devices showed two conductance states as a function of ultraviolet/Vis irradiation ( Fig. 4c ). The trans -isomer in the low-conducting state transforms into a cis -isomer in the high-conducting state, a process that involves short-distance tunnelling transport (h1>h2 in Fig. 4b ) in cis -aryl azobenzene molecular junctions [23] . The reversible photo-induced conformational changes of the aryl azobenzene monolayer were repeatedly plotted as the change in current density with respect to the switching number ( Fig. 4d ). Over more than 50 cycles of reversible photo-switching, the two conductance states were almost identical and reproducible, indicating that highly stable photo-switchable molecular monolayer devices were achieved using the novel type of graphene junction. In addition to photo-induced conductance switching, applied voltages can induce two molecular conductance states of the aryl azobenzene monolayer [24] . Furthermore, the voltage pulses of 3.0 V/−3.0 V ( Supplementary Fig. S12 ) caused the azobenzene molecules to reversibly transform between the trans -isomer and the cis -isomer, while the devices featuring aryl alkanes did not show voltage-induced molecular conductance switching at all. Also, the preservation test plots of device performances after bending the devices at a certain angle indicated that voltage-driven conformational changes between the two isomers occurred, showing the stability of the flexible molecular electronic devices. Consequently, the asymmetric junction structure with a chemical bottom contact and a physical top contact can effectively switch between the trans and cis -isomer conformations under applying voltages. 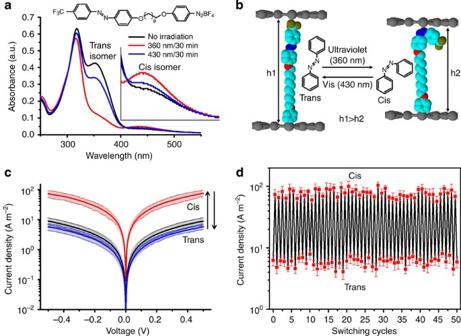Figure 4: Photo-switching of graphene-aryl azobenzene monolayer–graphene devices. (a) Chemical structure of aryl azobenzene and ultraviolet-Vis spectra in solution regarding ultraviolet/Vis irradiation. Inset shows the zoomed-in spectra at a range from 400 to 550 nm. (b) Molecular tunnelling barriers (with h1 and h2 being the vertical distance between the two graphene electrodes) corresponding to conformational changes in aryl azobenzene molecules with light irradiation. (c) Photo-induced current density-voltage plots on a log scale over a low voltage range for the graphene-aryl azobenzene monolayer–graphene devices. (d) Current density plots for each isomer state over 50 cycles of reversible photo-switching (induced by ultraviolet/Vis irradiation per 45 min); the plots were generated from average values obtained at 0.3 V from over five devices (the error bars denote the s.d. values obtained from over 20 data points for each state). Figure 4: Photo-switching of graphene-aryl azobenzene monolayer–graphene devices. ( a ) Chemical structure of aryl azobenzene and ultraviolet-Vis spectra in solution regarding ultraviolet/Vis irradiation. Inset shows the zoomed-in spectra at a range from 400 to 550 nm. ( b ) Molecular tunnelling barriers (with h1 and h2 being the vertical distance between the two graphene electrodes) corresponding to conformational changes in aryl azobenzene molecules with light irradiation. ( c ) Photo-induced current density-voltage plots on a log scale over a low voltage range for the graphene-aryl azobenzene monolayer–graphene devices. ( d ) Current density plots for each isomer state over 50 cycles of reversible photo-switching (induced by ultraviolet/Vis irradiation per 45 min); the plots were generated from average values obtained at 0.3 V from over five devices (the error bars denote the s.d. values obtained from over 20 data points for each state). Full size image Our work could lead to flexible devices applications of molecular electronics beyond conventional Si substrate- or metal electrode-based devices. Like metal electrodes, a graphene electrode served the chemically applicable surface to form molecular monolayers of molecules specified with an electrophilic group (for example, the dediazoniation process of diazonium molecules on graphene). Graphene, a single-layer of carbon atoms form ideal electrical contacts via formation of carbon-carbon bonding to organic molecules as ultimate materials for flexible electronics. The use of both the graphene electrodes in a two-terminal vertical device provides stable contacts to molecular monolayers, leading to high flexibility against mechanical stresses such as bending and twisting. Also molecular devices with the two graphene electrodes are electrically stabilized because of a metal-free process for electrical contacts on vulnerable molecular monolayers, preventing an electrical short circuit. High sensitivity of graphene to molecular functionalities gains advantages to realize molecular electronics beyond other metal electrodes. Moreover, two transparent and conductive graphene electrodes that make one-sided physically bound contacts to molecules in molecular monolayer devices enables to operate and transmit photo-induced changes in the molecular conformational length of aryl azobenzene molecules. In summary, self-assembly of aryl molecules on graphene was monitored by nanogravimetry. Molecular monolayer junctions between the two graphene electrodes were successfully fabricated and well-exhibited tunneling transport through molecular monolayers under the severe influences of bending and twisting. Photo-switchable aryl azobenzene monolayers between highly flexible and transparent graphene electrodes showed a stable device performance with a large number of reversible photo-switching cycles between trans -isomer at the low conductance and cis -isomer at the high conductance. Materials and characterization (I) Aryl diazonium salts (4-alkyl (for example, octyl, decyl and dodecyl)-benzenediazonium tetrafluoroborate) were synthesized according to previously reported methods [3] , [25] ( Supplementary Fig. S1 ). In a 50-ml round bottom flask, 4-alkyl (for example, octyl, decyl and dodecyl)-aniline (0.200 g) was dissolved in dry CH 2 Cl 2 (10 ml) under N 2 . This solution was added dropwise with a syringe to borontrifluoride etherate (2 equiv.) in a 100-ml round bottom flask cooled to −5 °C under N 2 . Isoamyl nitrite (1.6 equiv.) was then added dropwise to the mixture with a syringe and a solid subsequently formed. The mixture was allowed to stir for 30 min at −5 °C before it was warmed to room temperature. The solid was then filtered and the filter cake was washed with cold Et 2 O to yield a white-yellow solid after drying: characterization data for 4-octyl-benzenediazonium tetrafluoroborate; 1 H NMR (300 MHz, (C=O(CD 3 ) 2 ): δ 8.62 (d, J =9.0 Hz, 2H), 7.88 (d, J =8.7 Hz, 2H), 2.89 (t, J =7.7 Hz, 2H), 1.68 (m, 2H), 1.30 (m, 10H), 0.91(t, J =6.8 Hz, 3H); 13 C NMR (300 MHz, (C=O(CD 3 ) 2 ): δ 158.5, 133.2, 131.6, 112.6, 36.2, 31.7, 29.4. Characterization data for 4-decyl-benzenediazonium tetrafluoroborate; 1 H NMR (300 MHz, (C=O(CD 3 ) 2 ): δ 7.18 (d, J =8.1 Hz, 2H), 7.01 (d, J =8.1 Hz, 2H), 1.59 (m, 2H), 1.29 (m, 16H), 0.90 (t, J =6.5 Hz, 3H); 13 C NMR (300 MHz, (C=O(CD 3 ) 2 ): δ 162.0, 137.6, 129.6, 119.8, 34.9, 31.7, 29.5. Characterization data for 4-dodecyl-benzenediazonium tetrafluoroborate; 1 H NMR (300 MHz, (C=O(CD 3 ) 2 ): δ 7.06 (d, J =8.1 Hz, 2H), 6.87 (d, J =8.4 Hz, 2H), 1.49 (m, 2H), 1.22 (m, 20H), 0.84 (t, J =5.7 Hz, 3H); 13 C NMR (300 MHz, (C=O(CD 3 ) 2 ): δ 168.7, 137.4, 129.5, 119.3, 34.9, 31.8, 29.5. (II) Aryl azobenzene (AB) diazonium salts: (E)-4-(10-(4-((4-(trifluoromethyl)phenyl)diazenyl)phenoxy)decyloxy)benzenediazonium tetrafluoroborate was also synthesized and characterized as reported in a previous paper [25] ( Supplementary Fig. S2 ). (III) Single-layer CVD graphene on a Cu foil was supplied by the Graphene Center at Sungkyunkan University. The CVD graphene was transferred onto the substrates by the PMMA-mediated method, as described (or modified) in a previous paper [16] ; (1) spin-coating PMMA (~50 mg ml −1 in chlorobenzene) on graphene/Cu foil, (2) drying PMMA/graphene/Cu foil at 90 °C for 3 min (or under air blowing in a clean bench), (3) O 2 plasma etching of graphene on the backside of Cu foil, (4) wet-etching Cu foil floating in an ammonium persulfate solution (20 g l −1 in distilled water), (5) transferring and washing a PMMA/graphene sheet (more than two times) using an SiO 2 substrate with distilled water, (6) transferring a PMMA/graphene sheet onto appropriate substrates, (7) drying the PMMA/graphene/substrate under air in a clean bench, (8) removing PMMA with warm acetone (several times), (9) washing the graphene/substrate with isopropyl alcohol, (10) drying the graphene/substrate under air in a clean bench, followed by drying under vacuum. (IV) The CVD graphene was characterized by atomic force microscopy (Agilent 5,100 AFM/SPM system), TEM (JEOL JEM-2,100F), Fourier transform infrared (Bruker IFS-66/S), and Raman spectroscopy (Reinshaw, RM1,000-In Via). The self-assembly of the aryl diazonium compounds was monitored by a nanogravimetry technique (EQCN, Shin) using a graphene-covered quartz crystal resonator (formed on a gold-coated quartz crystal from International Crystal Manufacturing Co, Inc.). Cyclic voltammetry (CHI, Electrochemical Analyzer 660A) of the graphene was performed under inert conditions in a three-electrode electrochemical cell that consisted of a Pt-wire counter electrode, an Ag/AgCl reference electrode and a graphene-covered gold working electrode. Fabrication of molecular monolayer devices To construct the graphene-based molecular junctions, PDMS/PET substrates were patterned with Au(50 nm)/Ti(5 nm) leads by e-beam evaporation at a low deposition rate of 0.1 Å s −1 before transferring the graphene bottom electrode. The substrate was treated with O 2 plasma immediately before transferring the graphene bottom electrode to improve the surface wettability. After transferring the graphene bottom electrode, 20~70 mM of aryl diazonium compounds were dissolved in dimethylformamide (DMF) and then grafted onto the graphene-covered substrates by incubation in a glove box for 15~30 h. The aryl alkane or azobenzene monolayers on graphene were thoroughly washed with DMF and then dried overnight in a vacuum. After transferring the graphene top electrode on the monolayers, Au(50 nm) leads by e-beam evaporation at a low deposition rate of 0.1 Å s −1 . For the final active device area of 300 × 300 μm 2 ( Supplementary Fig. S3 ) extra graphene, the rest of graphene on the outside of the active device area was etched with O 2 plasma (50 W per 30 s and 100 W per 30 s, Cute/Femto Science) at each subsequent step after transferring graphene. The electrical characteristics of the devices were measured with a Keithley 4200-SCS semiconductor characterization system under ambient conditions. Ultraviolet-Vis spectroscopy was performed using a Shimadzu ultraviolet-3600 ultraviolet-Vis-NIR. Photo-irradiation with 360/430 nm light was performed using a Power Arc ultraviolet 100 instrument (ultraviolet Process Supply Inc.). How to cite this article: Seo, S. et al . Photo-switchable molecular monolayer anchored between highly transparent and flexible graphene electrodes. Nat. Commun. 4:1920 doi: 10.1038/ncomms2937 (2013).